Enamel-like apatite crown covering amorphous mineral in a crayfish mandible Carbonated hydroxyapatite is the mineral found in vertebrate bones and teeth, whereas invertebrates utilize calcium carbonate in their mineralized organs. In particular, stable amorphous calcium carbonate is found in many crustaceans. Here we report on an unusual, crystalline enamel-like apatite layer found in the mandibles of the arthropod Cherax quadricarinatus (freshwater crayfish). Despite their very different thermodynamic stabilities, amorphous calcium carbonate, amorphous calcium phosphate, calcite and fluorapatite coexist in well-defined functional layers in close proximity within the mandible. The softer amorphous minerals are found primarily in the bulk of the mandible whereas apatite, the harder and less soluble mineral, forms a wear-resistant, enamel-like coating of the molar tooth. Our findings suggest a unique case of convergent evolution, where similar functional challenges of mastication led to independent developments of structurally and mechanically similar, apatite-based layers in the teeth of genetically remote phyla: vertebrates and crustaceans. Teeth are exposed to considerable abrasion and mechanical stresses. The structure, mineralogy and composition of these mastication tools are intimately linked to feeding habits and are subject to evolutionary selective pressures. As a result, teeth are usually the hardest parts of the body, with superior wear-resistance and biomechanical toughness. Typically, a tooth can be divided into three structurally important components: a hard and wear-resistant working part, a softer supporting 'cushion' that can withstand the impacting, compressive or tensile stresses and a hard–soft interface that is usually mechanically graded to minimize interfacial stresses [1] , [2] , [3] . Diverse examples for the formation of this tri-element tooth structural approach are known. Among the mollusks, chitons (Polyplacophora) use iron oxide (magnetite) [4] , [5] along with calcium phosphate mineral [6] in their teeth while limpets (Gastropoda) form iron oxide (goethite) and silica-laden teeth [7] . The better-known calcium phosphate (hydroxyapatite)-based mammalian teeth, where a hard enamel layer covers a softer bulk of dentin to form highly efficient cutting and grinding tools [3] are of course a benchmark reference for teeth structure. Another interesting example are the self-sharpening sea urchin (Echinoidea) teeth with grinding tips that are made of calcite reinforced with high content of magnesium ions, to a level close to dolomite [8] , [9] . Common to all these teeth types is the choice, or compositional modification of minerals for increased hardness of the working surface [8] and the exquisite control of their location and ultrastructural organization. The latter is often characterized by fibrillar or elongated needle structures oriented perpendicular to the load bearing direction. Various designs are also found in the interfaces between the hard cover and the underlying softer support layer. A well-known example is the mammalian dentin–enamel junction, a distinct layer that prevents crack propagation from enamel into dentin [10] , [11] . An interesting alternative to all these highly mineralized teeth are the sclerotized teeth of Polychaete worms, where the use of mineral (copper biominerals) is sparse [12] , [13] and non-mineralized zinc and copper serve to crosslink and harden a proteinaceous matrix rich in histidine [13] , [14] . In the current study, we investigate the mandible of the arthropod Cherax quadricarinatus (freshwater crayfish). In crustaceans, the mandibles are part of the exoskeleton and are periodically removed and regenerated during each molting cycle that may occur every few days in early growth stages [15] . In contrast to mammalian bone and dentin, which are collagen-based tissues with embedded carbonated hydroxyapatite crystals, the exoskeletons of crustaceans are chitin-based and commonly reinforced with calcium carbonate [16] . The cuticle of C. quadricarinatus is known to contain amorphous calcium carbonate (ACC) [15] , [17] , which can be easily dissolved before the molting as compared with its crystalline polymorphs [15] , [18] . We found that the mandibles of the freshwater crayfish contain more than only ACC mineral. They are in part covered by a layer of fluorapatite (FAP) crystals, reminiscent of the hydroxyapatite-based enamel found in vertebrate teeth. We studied the crayfish mandibles on various length-scales and discovered that the complex functional tooth structure is quickly grown by carefully combining amorphous and crystalline minerals. The appearance of an enamel-like apatite layer and similarities in the investigated mechanical properties of the molar crayfish tooth and mammalian teeth suggest a unique case of convergent evolution. Similar functional challenges of needing to grind food, led to remarkably similar solutions that appeared independently in genetically remote phyla: the vertebrates and this ancient group of arthropods [19] . Four different minerals found in the mandible In crayfish, the mandibles form the anterior mouthparts, located directly in front of the oral opening ( Fig. 1a ). The mandibles consist of a large base, capped with two protuberances: the molar ridge, which serves as a massive grinding surface for mastication, and the incisor process, which serves for grabbing and holding food [20] ( Fig. 1b ). The anterior molar ridge of C. quadricarinatus contains a large tooth that is distinct from the rest of the mandible in both colour and form ( Fig. 1c ). Raman spectroscopy ( Fig. 1d ) revealed that the mandible contains four different minerals: ACC and amorphous calcium phosphate (ACP) in the base of the mandible, calcite in the incisor and, most surprisingly, FAP in the anterior molar. 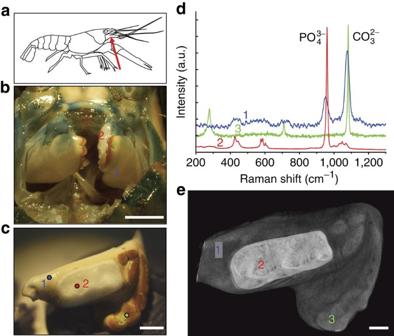Figure 1: Distribution of different minerals in the mandible. (a) Schematic representation of the crayfish (C. quadricarinatus), red arrow indicating the position of the oral opening. (b) Ventral view of the mandible and the oral opening showing the basal segment (1), the anterior molar (2) and the outer incisor (3). Scale bar, 5 mm. (c) Detailed view of an isolated mandible. The coloured points indicate positions where Raman spectra (shown ind) were measured. Scale bar, 2 mm. (d) Chemical analysis of the mandible by Raman spectroscopy reveals the coexistence of amorphous carbonate and phosphate in the basal segment (blue, broadened peaks), apatite in the molar (red) and calcite in the incisor (green). The calcite is located beneath the brown chitinous cover of the incisor whereas the molar apatite is exposed. The main mode (ν1) of carbonate and phosphate are indicated. (e) Micro-CT image of the mandible showing higher density of the molar tooth due to increased attenuation (brighter regions) of the molar with respect to the basal segment and anterior incisor. The scale bar corresponds to 1 mm. Figure 1e shows an X-ray tomography reconstruction of such a mandible. The significantly higher density of the molar (due to higher X-ray attenuation) corresponds to the bright appearance of the tissues observed in Fig. 1c . Figure 1: Distribution of different minerals in the mandible. ( a ) Schematic representation of the crayfish ( C. quadricarinatus) , red arrow indicating the position of the oral opening. ( b ) Ventral view of the mandible and the oral opening showing the basal segment (1), the anterior molar (2) and the outer incisor (3). Scale bar, 5 mm. ( c ) Detailed view of an isolated mandible. The coloured points indicate positions where Raman spectra (shown in d ) were measured. Scale bar, 2 mm. ( d ) Chemical analysis of the mandible by Raman spectroscopy reveals the coexistence of amorphous carbonate and phosphate in the basal segment (blue, broadened peaks), apatite in the molar (red) and calcite in the incisor (green). The calcite is located beneath the brown chitinous cover of the incisor whereas the molar apatite is exposed. The main mode (ν 1 ) of carbonate and phosphate are indicated. ( e ) Micro-CT image of the mandible showing higher density of the molar tooth due to increased attenuation (brighter regions) of the molar with respect to the basal segment and anterior incisor. The scale bar corresponds to 1 mm. Full size image The microstructure of the molar tooth Phase contrast-enhanced synchrotron-based X-ray microtomography revealed the 3D internal microstructure of the molar ( Fig. 2a ), combining the effects of density variations with contrast arising because of the diffraction of X-rays at interfaces within the specimen [21] . A virtual slice through the tomogram of a water-immersed typical tooth ( Fig. 2a ) highlights two different zones, namely the apatite high-density mineral layer (light grey, to the right) and the base of the mandible (medium grey, centre), consisting of lower-density chitin and amorphous mineral. The outermost grinding surface is found on the right hand side of the image (delineated by the white–black line caused by X-ray interference effect). The apatite layer contains an array of parallel channels arranged normal to the outer surface, in a radial direction. These channels are similar and analogous to the crustacean cuticular pore canal system that is formed by cellular extensions of the epithelial cells [22] . The channels cross the cuticular 'basal layer', running through the amorphous mineral/chitin bulk, gradually thinning out towards the surface and finally terminating below the external tooth surface. 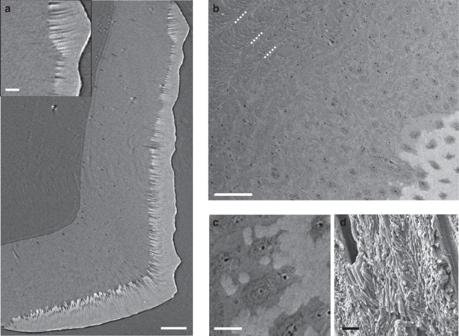Figure 2: Microstructure of the anterior molar. (a) Virtual slice perpendicular to the tooth working-surface (situated on the right) in a 3D phase contrast-enhanced synchrotron X-ray microtomography image. The external apatite layer (light grey) contains a complex 3D network of pore canals that interface with the underlying chitin and amorphous mineral-based jaw (medium grey). The inset shows a magnification of the apatite layer and the rough interface region with finger-like extensions. Scale bar, 100 μm. Inset scale bar, 20 μm. The spots and stripes in the dark-grey void on the left (beneath the inset, in the sample immersion liquid, with faint repeated patterns extending onto the mandible base) are ring artefacts, typical of high-resolution tomography. (b) SEM image (backscattered electrons) of a diagonal polished cross-section, showing the interface region between the apatite (bright) and the chitin tissue with amorphous mineral (dark grey). The white dotted lines indicate layers of a twisted plywood structure. Scale bar, 20 μm. (c) A magnification of the pore canals. The scale bar equals 5 μm. (d) SEM image (secondary electrons) of a fracture surface of the apatite layer. Large crystals are aligned in the direction of the canals. Scale bar, 2 μm. Figure 2b is a low-vacuum environmental scanning electron micrograph depicting a diagonal polished section of the transition zone between the apatite (bright on the lower right side) and the amorphous mineral reinforced chitin (dark). This section reveals typical details seen in cross-sectional slices at various depths beneath the outer surface. It is observed that the channels are situated about 6–8 μm apart, with the apatite mineralization beginning sparsely as isolated islands appearing between canals ( Fig. 2c ). Closer to the outer surface, apatite replaces the amorphous carbonate minerals in close proximity to the channels. The two mineral phases, the external apatite layer and internal chitin-amorphous mineral layer are interdigitated and form a convoluted interface. Conventional secondary electron scanning electron microscopy (SEM) of a fracture-surface ( Fig. 2d ) revealed elongated apatite crystals (typical size: 0.5 μm thickness ×3 μm length) oriented parallel to the pore canals direction. The 'grainy' matter seen surrounding the canals is presumably the amorphous mineral. Figure 2: Microstructure of the anterior molar. ( a ) Virtual slice perpendicular to the tooth working-surface (situated on the right) in a 3D phase contrast-enhanced synchrotron X-ray microtomography image. The external apatite layer (light grey) contains a complex 3D network of pore canals that interface with the underlying chitin and amorphous mineral-based jaw (medium grey). The inset shows a magnification of the apatite layer and the rough interface region with finger-like extensions. Scale bar, 100 μm. Inset scale bar, 20 μm. The spots and stripes in the dark-grey void on the left (beneath the inset, in the sample immersion liquid, with faint repeated patterns extending onto the mandible base) are ring artefacts, typical of high-resolution tomography. ( b ) SEM image (backscattered electrons) of a diagonal polished cross-section, showing the interface region between the apatite (bright) and the chitin tissue with amorphous mineral (dark grey). The white dotted lines indicate layers of a twisted plywood structure. Scale bar, 20 μm. ( c ) A magnification of the pore canals. The scale bar equals 5 μm. ( d ) SEM image (secondary electrons) of a fracture surface of the apatite layer. Large crystals are aligned in the direction of the canals. Scale bar, 2 μm. Full size image The distribution and orientation of mineral and chitin A polished cross-section through a crayfish molar tooth (light micrograph Fig. 3a ) was imaged by means of microbeam scanning wide-angle X-ray scattering (WAXS) measurements. The micro-diffractograms provided mineralogical identification, relative abundance and orientation information, presented for chitin ( Fig. 3b ), amorphous minerals ( Fig. 3c ) and apatite ( Fig. 3d ). Examples of typical diffraction patterns are shown for the mandible base ( Fig. 3e ), the transition ( Fig. 3f ) and apatite zones ( Fig. 3g ) of the organ. The positions of the measurements are indicated by circles in Fig. 3b–d . These patterns show a diffuse ring due to amorphous mineral, as well as chitin and apatite diffraction arcs that were used to derive the pictures presented in Fig. 3b–d . The apatite crystals are roughly co-aligned with their c -axes orthogonal to the outer surface throughout the entire apatitic layer. Two chitin fibrous components are observed: fibres running parallel to the molar tooth surface in the deeper layer, corresponding to the known cuticle 'twisted plywood' structure [23] (also delineated in Fig. 2b by dashed lines), and fibres preferentially oriented orthogonal to the surface [24] , running parallel to the channel radial direction in the region adjacent to the interface with the apatite (black lines in Fig. 3b showing the predominant chitin c -axis orientation changing close to the grinding surface). The amorphous mineral content increases towards the outer part of the tooth structure ( Fig. 3c ). 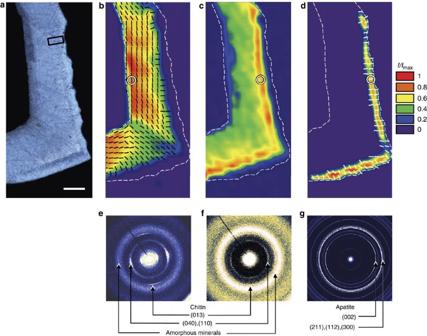Figure 3: Spatial distribution and orientation of chitin and mineral. (a) Light micrograph of a cross-section of the molar tooth used for synchrotron scanning WAXS measurements (entire region) and Raman imaging (black rectangle,Fig. 4). Scale bar, 200 μm. (b) Amount (colour code) and orientation (caxis, black lines) of chitin fibres. In the basal part, the layered plywood structure dominates, whereas, in the outer parts, the chitin fibres are predominantly oriented perpendicular to the tooth surface. (c) Normalized scattering intensity (colour code) of the amorphous mineral phase (ACC+ACP) showing increased amount and contrast towards the interface with the apatite. (d) Amount (colour code) and orientation (crystallographiccaxis, white lines) of FAP. These crystals are mainly oriented perpendicular to the surface. All 2D maps inb–dshow normalized integrated intensitiesI/Imax(peak area) and orientations of WAXS peaks of the different phases. The dashed white lines trace the contour of the tooth. (e) Example for a diffraction pattern obtained in the mandible base (position indicated by a circle inb). (f) Typical diffraction pattern for the transition zone (position indicated inc). (g) Diffraction pattern for the apatite zone (position indicated ind). Figure 3: Spatial distribution and orientation of chitin and mineral. ( a ) Light micrograph of a cross-section of the molar tooth used for synchrotron scanning WAXS measurements (entire region) and Raman imaging (black rectangle, Fig. 4 ). Scale bar, 200 μm. ( b ) Amount (colour code) and orientation ( c axis, black lines) of chitin fibres. In the basal part, the layered plywood structure dominates, whereas, in the outer parts, the chitin fibres are predominantly oriented perpendicular to the tooth surface. ( c ) Normalized scattering intensity (colour code) of the amorphous mineral phase (ACC+ACP) showing increased amount and contrast towards the interface with the apatite. ( d ) Amount (colour code) and orientation (crystallographic c axis, white lines) of FAP. These crystals are mainly oriented perpendicular to the surface. All 2D maps in b – d show normalized integrated intensities I / I max (peak area) and orientations of WAXS peaks of the different phases. The dashed white lines trace the contour of the tooth. ( e ) Example for a diffraction pattern obtained in the mandible base (position indicated by a circle in b ). ( f ) Typical diffraction pattern for the transition zone (position indicated in c ). ( g ) Diffraction pattern for the apatite zone (position indicated in d ). Full size image The distribution of carbonate and phosphate The local chemical composition along the tooth section was studied by Raman spectroscopic imaging and the data are presented in Fig. 4 (a second region is given in the Supplementary Fig. S1 ). The position of the analysed region (light micrograph shown in Fig. 4a ) with respect to the WAXS measurements is indicated by the black rectangle in the light micrograph in Fig. 3a . The images in Fig. 4b–d show the intensities of the phosphate band ( Fig. 4b ), the carbonate-to-phosphate ratios ( Fig. 4c ) and the shifts of the centre-of-mass of the phosphate peak ( Fig. 4d ). Phosphate is found within the entire measured region extending from the apatite layer deep into the amorphous mineral, with a strong gradient at the interface between the bulk of the molar and the outer apatite layer ( Fig. 4b ). The carbonate/phosphate ratio shows a pronounced gradient even within the amorphous mineral phase, far from the molar surface, with several fluctuations ( Fig. 4c ) that may reflect temporal physiological variations at the time of deposition. The phosphate ν 1 peaks around 950–965 cm −1 consist of two, partially overlapping peaks, that is, a sharper peak at 965 cm −1 of the FAP covering layer, and a broader peak centred at 951 cm −1 of the underlying ACP rich layer. The shift in peak position is the outcome of a gradual increase in FAP near the transition zone, ( Fig. 4a (sampling pts 2–5) and Fig. 4e ). The abrupt transition seen in Fig. 4d marks the line where FAP abundance overrides ACP. Indeed, the shift to lower wavenumbers is associated with a broadening of the carbonate and phosphate ν 1 vibrational modes (as compared with calcite and FAP standards, Fig. 4e ), and is characteristic of an amorphous, disordered mineral phase [25] , [26] . According to Fig. 4c , the carbonate content in the crystalline apatite is negligible but dominant in the underlying ACC/ACP layer, where both minerals coexist. Moreover, the position of the phosphate band in the Raman spectrum of the apatite region of the tooth corresponds to a band shift usually associated with high fluoridation of apatite [27] . High-resolution powder X-ray diffraction measurements ( Supplementary Fig. S2 ) and Energy dispersive spectroscopy (EDS) analysis ( Supplementary Table S1 ) further corroborate that the crayfish molar is covered by FAP. 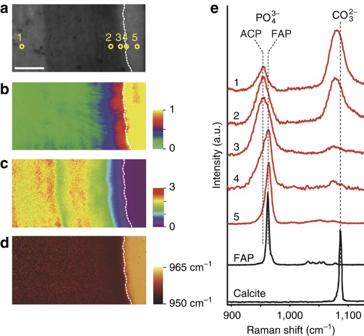Figure 4: Raman spectroscopic imaging of the anterior molar. (a) Light micrograph of the analysed area. Scale bar, 20 μm. The measured area on a cross-section covers the transition zone between the apatite and the amorphous mineral and is indicated by the black rectangle in the light micrograph shown inFig. 3a. (b) Raman spectroscopic image of the ν1phosphate peak. The normalized integrated intensity () illustrates that phosphate is found in the entire mapped region. (c) The intensity ratio () of the carbonate (ν1) to the phosphate peak shows a pronounced gradient with superimposed fluctuations. (d) The position of the ν1phosphate peak shows a transition between the predominance of the crystalline (higher values) and the amorphous regions (lower values). The boundary between the apatite layer and the amorphous phases is indicated by the white dashed lines inb–d. (e) Normalized single Raman spectra at positions 1, 2, 3, 4 and 5 as indicated ina, compared with synthetic reference materials (FAP and calcite). The changes in the peak intensities show the gradual decrease/increase in carbonate/phosphate amount. The broadening of the phosphate peak as well as the shift to lower wavenumbers, when passing from position 5 to position 3 across the sample, can be seen. Figure 4: Raman spectroscopic imaging of the anterior molar. ( a ) Light micrograph of the analysed area. Scale bar, 20 μm. The measured area on a cross-section covers the transition zone between the apatite and the amorphous mineral and is indicated by the black rectangle in the light micrograph shown in Fig. 3a . ( b ) Raman spectroscopic image of the ν 1 phosphate peak. The normalized integrated intensity ( ) illustrates that phosphate is found in the entire mapped region. ( c ) The intensity ratio ( ) of the carbonate (ν 1 ) to the phosphate peak shows a pronounced gradient with superimposed fluctuations. ( d ) The position of the ν 1 phosphate peak shows a transition between the predominance of the crystalline (higher values) and the amorphous regions (lower values). The boundary between the apatite layer and the amorphous phases is indicated by the white dashed lines in b – d . ( e ) Normalized single Raman spectra at positions 1, 2, 3, 4 and 5 as indicated in a , compared with synthetic reference materials (FAP and calcite). The changes in the peak intensities show the gradual decrease/increase in carbonate/phosphate amount. The broadening of the phosphate peak as well as the shift to lower wavenumbers, when passing from position 5 to position 3 across the sample, can be seen. Full size image The mechanical properties of the molar tooth The mechanical properties of a molar tooth cross-section ( Fig. 5a ) were tested by nanoindentation ( Fig. 5b ). We found that the hardness systematically changes from 4.5–5 GPa in the outer apatite layer to about 1 GPa in the base of the mandible that consists of chitin and amorphous mineral. A typical scan is plotted in Fig. 5b (open triangles), where a small gradient from about 1–2 GPa is seen in the base of the mandible reflecting the increase in amorphous mineral content, before the values sharply increase at the interface with the FAP layer. Hardness values in the FAP layer are significantly higher than what was previously reported for insect mandibles (3 GPa) [28] although the hardness of the base of the mandible is in the range (although slightly larger) of what was found in the crushing part of the lobster claw (0.5 GPa) [29] . The observed hardness profile is also remarkably similar to that of mammalian teeth [30] , which consist of dentin, with a hardness of about 0.7 to 1 GPa (refs 31 , 31 ) and enamel, with reported hardness values ranging from 3–6 GPa, depending on the direction of the nanoindentation [32] and position [33] in the tooth. The reduced moduli of the crayfish molar, evaluated from the unloading curves of the nanoindentation, follow the same trend as the hardness ( Fig. 5b , full circles). The apatite layer is on average more than three times as stiff and four times as hard as the underlying composite of chitin and amorphous mineral ( Table 1 ). 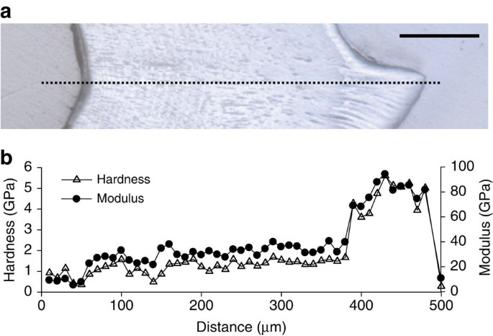Figure 5: Nanoindentation of the anterior crayfish molar. (a) Light micrograph of the measured region on a cross-section. Scale bar, 100 μm. (b) Hardness (open triangles) and reduced modulus (filled circles) for the dotted line ina. Both properties show an increase towards the apatite layer and much larger values within the FAP than in the chitin reinforced with amorphous mineral. Figure 5: Nanoindentation of the anterior crayfish molar. ( a ) Light micrograph of the measured region on a cross-section. Scale bar, 100 μm. ( b ) Hardness (open triangles) and reduced modulus (filled circles) for the dotted line in a . Both properties show an increase towards the apatite layer and much larger values within the FAP than in the chitin reinforced with amorphous mineral. Full size image Table 1 Nanoindentation of the molar tooth. Full size table The nanoindentation measurements of the crayfish molar were performed on a dry sample and are therefore correlated to, but may not precisely reflect the properties of the teeth in their hydrated natural state [29] . However, the mechanical properties of mineralized cuticle, and especially the densely mineralized crustaceans mouthparts are dominated by their constituent minerals and are therefore less susceptible to the effects of dehydration [34] , [35] . Hence our measurements are probably in fair agreement with their natural state. Our results show that the molar of C. quadricarinatus is a highly complex organ that possesses a range of interesting functional features, including the three dental elements of hard cover, soft support, and graded interface between these layers. The observed similarities in hardness values between the crayfish molar and mammalian teeth exist despite the very different mineralogical composition of the supporting material (chitin and amorphous minerals vs collagen and hydroxyapatite), the very remote taxonomic context and the different diets processed by the two types of teeth. Most interestingly, the hard outer layer of the molar crayfish tooth is composed of highly crystalline FAP prisms, oriented normal to the surface, along the co-oriented pore canals and parallel to the load direction. This structural solution for the formation of a hard, wear-resistant surface is remarkably similar to the solution evolved in vertebrates' enamel, which consists of oriented bundles of elongated hydroyapatite crystals. The concept of reinforcing the outermost layer of a tooth with oriented, elongated crystals is relatively widespread. Nevertheless, the different examples described in the introduction show that many invertebrates have evolved completely different solutions based on a variety of minerals and other components. Importantly, from an evolutionary perspective, the appearance of such highly crystalline apatite in crustacean teeth is unexpected. Apatite is commonly well documented in two evolutionary groups: the Chordate (vertebrates) and a small class of invertebrates from the brachiopods (Lingulata) [36] . The crustaceans, like most of the invertebrates use calcium carbonate for exoskeleton reinforcement. A few exceptions of apatite formation in invertebrates were reported [6] , [37] . However, the apatite found in these invertebrates is nanocrystalline and is reminiscent of lamellar bone [37] . Remarkably, despite the great taxonomic distance, the crayfish molar apatite layer is composed of large apatite crystals, oriented parallel to the load direction, comparable in their mechanical performance to vertebrates' enamel [30] , [32] . The use of FAP in the crayfish molar as opposed to hydroxyapatite in mammalian teeth presumably is of advantage for the crustacean. FAP differs from hydroxyapatite only in the substitution of hydroxyl groups by fluorides [38] , yet has similar mechanical properties [27] . Fluoridation was previously also reported in the enameloid apatite of sharks [39] , [40] . Because of a lower water solubility [41] , [42] , the fluoridation of apatite presumably increases the durability of the teeth of C. quadricarinatus , which are mostly in contact with fresh water, rather than saliva as in mammals. The hard crown is mounted on a softer base of parallel oriented lamellar chitin reinforced with ACC, the typical structure of the crustacean exoskeleton. ACC is widely used in crustacean cuticles, presumably because of its high solubility. This property facilitates the periodic dissolution of the mineral before each molting cycle [15] . Besides ACC, many crustaceans also use calcite to reinforce their exoskeletons. However, the coexistence of a crystalline apatite forming the grinding surface with the underlying ACP-/ACC- graded interphase layer is reported here for the first time. Between the crystalline fluoroapatite crown and the soft ACC support, the mineral composition continuously transforms from ACP to ACC. The composition gradient is related directly to the variations in mechanical properties forming a unique type of graded interface. The combined structure of apatite and ACC is a physiological cost-effective solution where the metabolically 'expensive' and less resorbable phosphate is restricted to the outer surface whereas the resorbable 'common' carbonate is used for the bulk of the mandible and the cuticle. In conclusion, the molar of C. quadricarinatus is a highly complex, periodically renewable organ in which a unique architecture of amorphous and crystalline calcium carbonate and phosphate minerals constitutes a tooth with mechanical properties comparable to mammalian teeth. This is achieved by including gradients in the chemical composition and microstructure combining a highly crystalline apatite cap, reminiscent of enamel, covering a chitin scaffold reinforced with amorphous mineral. The similarities in their properties and underlying structural principles make the crayfish molar and mammalian teeth an interesting example of convergent evolution of a functional tooth structure based on hypermineralized enamel, which has been described as a 'masterpiece of bioceramics' [43] . Animals C. quadricarinatus crayfish were reared in artificial ponds at Ben-Gurion University, Beer-Sheva, Israel. The animals were anaesthetized in ice-cold water before dissection. Mature teeth were extracted from specimens at an inter-molt stage. SEM experiments were carried out with these as well as with exuvia samples. Ben-Gurion University Ethics Committee has exempted experiments with crustaceans from specific permit requirements Sample embedding and polishing Mandibles were kept frozen except during preparation to suppress any possible crystallization of amorphous minerals. Mandibles were embedded in Epofix cold-setting resin with a resin/hardener mixing ratio ( w / w ) of 25/3, and then sectioned with a slow diamond saw (BUEHLER Isomat, Germany) using petroleum distillate (BUEHLER Isocut fluid) as cooling fluid, because ACC is highly water soluble. Mandible sections were further polished using ethyleneglycol lubricant to reduce thickness and provide a flat surface for Raman imaging and Nanoindentation measurements. Raman spectroscopy and imaging Raman spectra reported in Fig. 1d were acquired on a Jobin-Yvon LabRam HR 800 micro-Raman system equipped with a liquid nitrogen cooled detector. A He–Ne laser source (633 nm), a ×50 microscope objective, a 100-μm confocal aperture and a 600-mm −1 grating were used, giving a resolution of 2–4 cm −1 . For Raman spectroscopic imaging, a confocal Raman microscope (CRM200, WITec, Ulm, Germany) equipped with a piezo-scanner was used (P-500, Physik Instrumente, Karlsruhe, Germany) with a ×60 (0.8 NA) objective and a diode-pumped 785-nm near-infrared laser (Toptica Photonics AG, Graefelfing, Germany, laser power 10 mW). The surface was scanned using 500 nm steps, and full spectra for each pixel were acquired (0.1 s integration time) with a thermoelectrically cooled CCD detector (DU401A-BV, Andor, UK) placed behind a grating (300 mm −1 ) spectrograph (Acton, Princeton Instruments, Trenton, NJ, USA) with a spectral resolution of ~6 cm −1 . For spectra in Fig. 4e , 1,200 mm −1 grating (UHTS 300, WITec, spectral resolution ~2 cm −1 ) and 5 s integration times were used. Laser power (10 mW full beam power at the sample) was adjusted to attain a sufficient signal-to-noise ratio and to avoid sample damage. The ScanCtrlSpectroscopyPlus software (version 1.38, WITec) was used for measurements and WITec Project Plus (version 2.02, WITec) for spectra processing. The phosphate and carbonate images were generated by integrating the intensity of the signal for the wavenumber ranges of phosphate (920–990 cm −1 ) and carbonate (1040–1125 cm −1 ). The phosphate band position reported in Fig. 4d was obtained using a centre-of-mass filter to calculate the intensity-weighted spectral position of the 920–990 cm −1 wavenumber range. Micro-tomography Molar-containing segments of the mandible were imaged using two microtomogaphy instruments: (a) a laboratory instrument (Skyscan 1072, Skyscan, Kontich, Belgium) operated at 100 keV and magnified to obtain a resolution of 6.5 μm ( Fig. 1e ). Data were reconstructed using the standard Nrecon reconstruction package (Skyscan) and the reconstructed volumes were visualized or virtually sliced to reveal the internal microstructure (Amira 5.2, Visage Imaging GmbH, Germany). (b) The high-resolution microtomography set-up of the BAMline at BESSY-II storage ring (Helmholtz-Zentrum Berlin, Germany), operated as described elsewhere [44] ( Fig. 2a ). For our samples, we used an energy of 30 keV and 1,200 projections were obtained spanning 180° around the rotation axis. An effective pixel size of 2.2 μm was used, and the detector system was positioned 150 mm behind the sample. The tomographic datasets were reconstructed using the European Synchrotron Radiation Facility program PyHST [45] and visualized as mentioned in (a) above. Scanning electron microscopy Dried molar teeth were fractured perpendicular to the molar surface, sputter-coated with gold and examined using a JEOL JSM-7400f electron microscope. Slices and polished samples were imaged uncoated in an FEI Quanta 600 using the low-vacuum mode of imaging by the large field gaseous secondary electrons detector, with an acceleration voltage of 2–4 kV. Microbeam WAXS Scanning WAXS measurements were performed at the μ-Spot beamline [46] (BESSY II storage ring, Helmholtz-Zentrum Berlin). Embedded cross-sections of the molar tooth were scanned with a step size of 50 μm using an energy of 15 keV, while collecting two-dimensional diffraction patterns. The local amount of chitin, amorphous mineral and apatite, visualized in the images in Fig. 3b–d , show the integrated intensities of the isolated orthogonal WAXS peaks of the respective phases of chitin and apatite, and of the diffuse scattering halo for the amorphous phase, in a pseudocolour. These maps provide direct visualization of the spatial distribution of these phases [47] . The orientation representation of the c-axes of apatite and chitin were obtained from the azimuthal maxima of the apatite (002), and chitin (013) reflection (see ref. 23 ) in the 2D diffraction patterns. These maxima allow us to determine the planes in which the crystallographic c -axes and the related morphological orientations lie. For apatite, the orientation of the c -axis shows the preferred alignment of the crystals. For chitin, it corresponds to the fibre's orientation. As two chitin fibre orientations within the volume were observed, only the one corresponding to the highest peak was used in the present evaluation and was attributed to the predominant local fibre orientation. Nanoindentation Nanoindentation was carried out in ambient conditions using an Ubi nanoindentation instrument (Hysitron) with a Berkovich diamond tip. To obtain hardness and reduced modulus, all load–displacement curves were analysed, using the method described by Oliver and Pharr [48] . 550 indentations were performed using a maximal load of 5,000 μN across the polished surface. A dwell time of 60 s was applied at peak load to take creep behaviour into account. Relatively large lateral steps of 10 μm between each indentation were used. Thus, plastically deformed zones from previous indentations did not affect our measurements. The effect of topography was minimized by finely polishing the sample surface (see sample embedding and polishing ). How to cite this article: Bentov, S. et al . Enamel-like apatite crown covering amorphous mineral in a crayfish mandible. Nat. Commun. 3:839 doi: 10.1038/ncomms1839 (2012).